Earthworms facilitate carbon sequestration through unequal amplification of carbon stabilization compared with mineralization A recent review concluded that earthworm presence increases CO 2 emissions by 33% but does not affect soil organic carbon stocks. However, the findings are controversial and raise new questions. Here we hypothesize that neither an increase in CO 2 emission nor in stabilized carbon would entirely reflect the earthworms’ contribution to net carbon sequestration. We show how two widespread earthworm invaders affect net carbon sequestration through impacts on the balance of carbon mineralization and carbon stabilization. Earthworms accelerate carbon activation and induce unequal amplification of carbon stabilization compared with carbon mineralization, which generates an earthworm-mediated ‘carbon trap’. We introduce the new concept of sequestration quotient to quantify the unequal processes. The patterns of CO 2 emission and net carbon sequestration are predictable by comparing sequestration quotient values between treatments with and without earthworms. This study clarifies an ecological mechanism by which earthworms may regulate the terrestrial carbon sink. Biotic interactions between soil invertebrates and microbiota have essential roles in regulating land–atmosphere exchanges of carbon (C) and carbon-cycle feedbacks on climate change [1] . A timely topic is how earthworms interact with microbiota and, thus, affect C sequestration [2] , [3] , [4] . A recent meta-analysis suggested that earthworms increase CO 2 emissions by 33% but do not affect soil organic carbon (SOC) stocks as compared with treatments without earthworms [5] . However, this study raises four questions: First, why did earthworms belonging to different functional groups stimulate similar CO 2 emissions? Second, why did the earthworm-induced CO 2 emissions decrease with the extension of experimental period? Third, what caused the stimulated CO 2 emissions to be relatively less important in C-rich soil? And finally, why did SOC stocks not decrease if earthworms continuously stimulate CO 2 emissions [6] , [7] , [8] ? These puzzles may arise because C mineralization (C min ) and C stabilization (C sta ; refs 9 , 10 ) are usually studied separately. In general, C mineralization and C stabilization are coupled and closely related processes [11] . For a system without earthworms, soil microbiota themselves will activate (C activation; C act ) potentially mineralizable C (PMC) (C act-m ) at a basal rate, and convert it into readily mineralizable C (C min-m, that is, C basal-m ) and stabilized C (C sta-m ), that is, C act-m =C min-m +C sta-m ( Fig. 1 ). In a system with earthworms, earthworms may metabolize and stabilize a proportion of the basal C (C basal-m ); further, earthworms and their gut microbiota may accelerate the activation of PMC to some extent (C act-w ; ref. 12 ), and also convert this newly activated C into readily mineralizable C and stabilized C, that is, C act-w +C basal-m =C min-w +C sta-w ( Fig. 1 ). Consequently, earthworms may reduce the pool size of PMC and increase the pool sizes of both readily mineralizable C and stabilized C. Therefore, for a given system, no matter whether earthworms are present or not, an increase in C mineralization (C min ) and C stabilization (C sta ) may be a natural consequence of an increased pool of activated carbon (C act ). The pool size of the activated C (C act ) and its allocation pattern into C mineralization (C min ) and C stabilization (C sta ) then determine the net C sequestration ( Fig. 1 ). 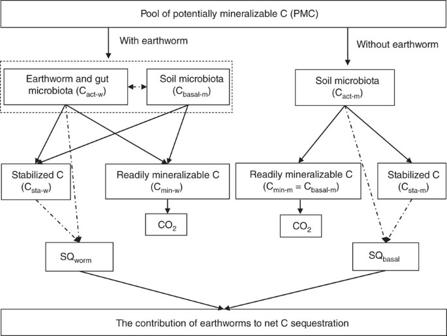Figure 1: Conceptual model of how earthworms regulate C sequestration. Cact-wand Cact-mrefer to the earthworm-activated and soil microbiota-activated mineralizable C, respectively. Cmin-wand Csta-wrefer to the net earthworm-induced pool of readily mineralizable C and pool of stabilized C in soil with earthworms, respectively; Cmin-mand Csta-mrefer to the pool of readily mineralizable C and pool of stabilized C, respectively, in soil without earthworms. Given that the soil microbiota-induced readily mineralizable C (Cmin-m) may also be metabolized and/or stabilized by earthworms, Cmin-mis also defined as basal C (Cbasal-m). Note that the value of Cmin-m(Cbasal-m) in a system with and without earthworms may gradually differ as earthworm incubation proceeds. Csta-wand Cact-ware the differences between Cstaand Cstaplus Cminbetween soil with and without earthworms, respectively. SQwormand SQbasalrefer to the C sequestration quotient in soil with and without earthworms, respectively. The single-ended dot-dash lines represent the major components for the calculation of SQ values. The double-ended dotted-line indicates possible interactions. Figure 1: Conceptual model of how earthworms regulate C sequestration. C act-w and C act-m refer to the earthworm-activated and soil microbiota-activated mineralizable C, respectively. C min-w and C sta-w refer to the net earthworm-induced pool of readily mineralizable C and pool of stabilized C in soil with earthworms, respectively; C min-m and C sta-m refer to the pool of readily mineralizable C and pool of stabilized C, respectively, in soil without earthworms. Given that the soil microbiota-induced readily mineralizable C (C min-m ) may also be metabolized and/or stabilized by earthworms, C min-m is also defined as basal C (C basal-m ). Note that the value of C min-m (C basal-m ) in a system with and without earthworms may gradually differ as earthworm incubation proceeds. C sta-w and C act-w are the differences between C sta and C sta plus C min between soil with and without earthworms, respectively. SQ worm and SQ basal refer to the C sequestration quotient in soil with and without earthworms, respectively. The single-ended dot-dash lines represent the major components for the calculation of SQ values. The double-ended dotted-line indicates possible interactions. Full size image Given that most of the ingested soil and litter are egested in casts [12] , [13] , [14] , earthworms likely metabolize only the PMC or basal C (C basal-m ). These forms of C can be mineralized by soil microbiota alone at a slightly slower rate. Hence, the size of both C act-m and C act-w will be restricted by the supply of PMC and thus, may not differ significantly ( Fig. 1 ). This suggests that the enhancement of CO 2 emission by earthworms (C min-w ) may be overestimated. In contrast, the effects of earthworms on C stabilization (C sta-w ) may be underestimated. A 14-year field study, which reported that earthworms decreased soil carbon storage by 600 kg per ha per year, appears to provide solid evidence that earthworms continuously reduce carbon storage [15] . However, this result may need to be re-considered. The soil carbon was actually reduced only during the first 2 years of earthworm invasion and was, then, maintained at a new equilibrium in subsequent years. Thus, this work may simply be an example of an earthworm-induced initial increase of CO 2 emission in the field. On the other hand, unlike the readily detected C mineralization, an increase in C stabilization is difficult to observe directly due to the strong background of soil C. Thus, the magnitudes of C stabilization have to be estimated indirectly by their negative effect on C mineralization. Most studies to date were conducted over study periods that apparently were too short for C stabilization (and its negative effect on C mineralization) to be detected and it may often be overlooked. For instance, the endogeic species ( Octolasion tyrtaeum ) reduced CO 2 production by 15–39% only in studies exceeding 100 days [7] , [16] , [17] . In addition, the earthworm-stabilized C (C sta-w ) in field environments has not been properly quantified because most studies are restricted to soil depths of 0–30 cm (refs 1 , 18 , 19 , 20 ); but the stabilized C may be re-distributed throughout the whole soil profile or even be transferred into ground water. Given that the earthworm-mediated aggregation processes may ‘trap’ activated C successfully [21] , we propose that earthworms may enhance C stabilization to a greater extent than C mineralization. If so, the greater the proportion of PMC activated by earthworms, the greater the proportion of PMC that may be stabilized. Here we perform a two-phase experiment to compare the C mineralization capacity of earthworms and soil microbiota, and then evaluate the impacts of earthworms on the balance of C mineralization and C stabilization. The comparatively soil-preferring Asian Amynthas agrestis and litter-preferring European Lumbricus rubellus are used to establish distinct interactive systems of earthworm and microbiota [22] . Our data reveal that earthworms accelerate soil C mineralization, but do not increase the total amount of C mineralized compared with soil microbiota alone; in contrast, earthworm presence significantly enhances soil C stabilization. The earthworm-generated unequal C processes are manifested in changes of C distribution among aggregate fractions and of the respective humification intensity. We introduce the new concept of sequestration quotient (SQ, C sta /C act ) to quantify the unequal C processes, and establish a theoretical framework to clarify an ecological mechanism by which earthworms may regulate the terrestrial C sink. C mineralization capacities of earthworm and microbiota The net C loss patterns during the two-phase experiment ( Fig. 2 ) suggested that earthworms accelerated soil C mineralization, but did not increase the total amount of C mineralized compared with soil microbiota alone. During the first 23 days of the experiment (phase I), SOC content declined in treatment with either A. agrestis ( t =−6.436, P =0.023) or L. rubellus ( t =−8.215, P =0.014) but was unchanged in the control (no earthworms) soil ( t =0.079, P =0.944) compared with the initial SOC content of field soil. The SOC content of the control soil declined significantly ( t =−9.124, P =0.012) after an additional 31 days of incubation (phase II), but stayed the same for A. agrestis -worked soil (Asoil) and L. rubellus -worked soil (Lsoil) from which earthworms had been removed before the start of phase II. Earthworms affected the coefficient of variation of SOC content in similar patterns. Consequently, at the end of the two-phase experiment (54 days), SOC content in the control soil decreased to a level similar to that in soils that had been incubated with earthworms for 23 days during phase I ( F =2.37, P =0.174). 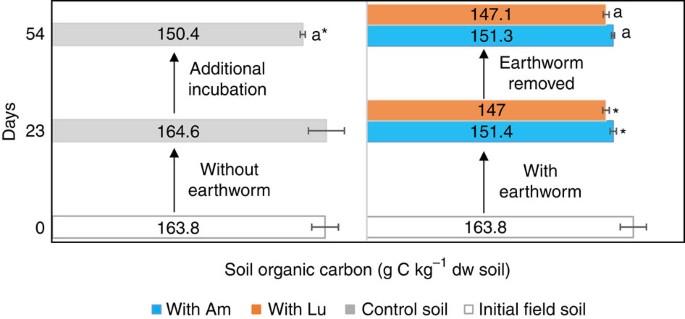Figure 2: Net loss of SOC compared with the initial field soil. Phase I: Sieved field soil (white block) was incubated with (coloured blocks) and without (control; grey block) earthworms for 23 days. Earthworms:L. rubellus(Lu; orange block),A. agrestis(Am; light blue block). Phase II: The incubated control soil and the two newly obtained earthworm-worked soils were incubated for an additional 31 days after removing earthworms. Values inside the boxes are the mean of SOC content (g C kg−1dw soil), with±1 s.e.m. indicated by error bars. A one-samplet-test (two-tailed) was performed between the mean organic C content of the initial field soil (n=9) and the SOC content of the field soil with and without earthworm incubation (n=3) after 23 days and again after further 31 days incubation; bars marked with ‘*’ indicate significant decline of soil C content compared with the mean C content of the initial field soil with date for a given treatment. A one-way ANOVA was performed to examine the differences among the control soil and the two earthworm-worked soils (that is, Asoil and Lsoil;n=3) at the end of phase II; bars marked with the letter ‘a’ indicate non-significant (P>0.05) differences of soil C content among treatments at day 54. Figure 2: Net loss of SOC compared with the initial field soil. Phase I: Sieved field soil (white block) was incubated with (coloured blocks) and without (control; grey block) earthworms for 23 days. Earthworms: L. rubellus (Lu; orange block), A. agrestis (Am; light blue block). Phase II: The incubated control soil and the two newly obtained earthworm-worked soils were incubated for an additional 31 days after removing earthworms. Values inside the boxes are the mean of SOC content (g C kg −1 dw soil), with±1 s.e.m. indicated by error bars. A one-sample t- test (two-tailed) was performed between the mean organic C content of the initial field soil ( n =9) and the SOC content of the field soil with and without earthworm incubation ( n =3) after 23 days and again after further 31 days incubation; bars marked with ‘*’ indicate significant decline of soil C content compared with the mean C content of the initial field soil with date for a given treatment. A one-way ANOVA was performed to examine the differences among the control soil and the two earthworm-worked soils (that is, Asoil and Lsoil; n =3) at the end of phase II; bars marked with the letter ‘a’ indicate non-significant ( P> 0.05) differences of soil C content among treatments at day 54. Full size image Balance of C mineralization and C stabilization The 23 days of earthworm incubation significantly enhanced soil C stabilization. Although similar amounts of C had been mineralized in all three treatments by the end of phase II ( Fig. 2 ), the remaining C in Asoil or Lsoil was more stable relative to that in the control soil ( Fig. 3a,b ). At this time, not only less SOC-derived CO 2 was emitted from Asoil ( P =0.033) and Lsoil ( P =0.076) ( Fig. 3a ) but also less litter-derived CO 2 was emitted from Asoil ( P <0.001) and Lsoil ( P =0.001) ( Fig. 3b ) as compared with the fluxes from the control soil. These results suggest that significant C stabilization accompanies transient earthworm-induced intensive C mineralization. The transient nature of the higher initial CO 2 emission in phase II also suggested that the magnitudes of earthworm-induced C mineralization were limited, and seemed to have already been damped by the process of earthworm-induced C stabilization. In phase II, L. rubellus and A. agrestis stimulated SOC- and litter-derived CO 2 only in the first and second week, respectively; and these effects were never significant in Asoil ( Fig. 3c,d ) in which less PMC may remain ( Fig. 3a,b ). Moreover, the distinct dietary patterns of the two earthworm species did not result in a significant difference in SOC- or litter-derived CO 2 emissions ( P =0.123 and P =0.938, respectively; n =6, repeated measures ANOVA). Therefore, earthworm biological traits such as dietary niche may not have a great impact on the magnitude of earthworm-induced C mineralization over the short term; in contrast, these traits may reduce C availability and, thus, the consequent C mineralization over the long term via regulating the magnitude of C stabilization. 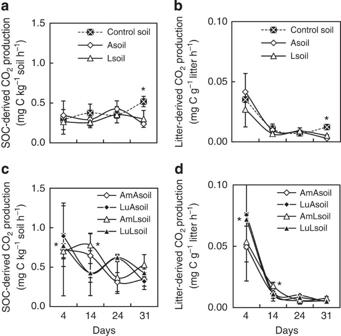Figure 3: Earthworm effects on carbon mineralization during phase II. SOC- and litter-derived CO2production from treatments without earthworms (control soil, Asoil and Lsoil; (a,b)) and with earthworms (c,d). In all panels, mean values are shown±1 s.e.m. (n=3); the s.e.m. is indicated by error bars. Asoil:A. agrestis-worked soil; Lsoil:L. rubellus-worked soil. ‘*’ indicates higher CO2emission from control soil than earthworm-worked soils at the end of phase II (panelsa,b), and indicates higher SOC- and litter-derived CO2emission from Lsoil withL. rubellusat day 4 or from Lsoil withA. agrestisat day 14 than those from Lsoil without earthworms (panelsc,d). At day 4,L. rubellusincreased SOC- and litter-derived CO2emission from Lsoil significantly withP=0.039 andP=0.05, respectively; while,A. agrestisincreased SOC- and litter-derived CO2emission from Lsoil significantly at day 14 withP=0.02 andP=0.026, respectively. Figure 3: Earthworm effects on carbon mineralization during phase II. SOC- and litter-derived CO 2 production from treatments without earthworms (control soil, Asoil and Lsoil; ( a , b )) and with earthworms ( c , d ). In all panels, mean values are shown±1 s.e.m. ( n =3); the s.e.m. is indicated by error bars. Asoil: A. agrestis -worked soil; Lsoil: L. rubellus -worked soil. ‘*’ indicates higher CO 2 emission from control soil than earthworm-worked soils at the end of phase II (panels a , b ), and indicates higher SOC- and litter-derived CO 2 emission from Lsoil with L. rubellus at day 4 or from Lsoil with A. agrestis at day 14 than those from Lsoil without earthworms (panels c , d ). At day 4, L. rubellus increased SOC- and litter-derived CO 2 emission from Lsoil significantly with P =0.039 and P =0.05, respectively; while, A. agrestis increased SOC- and litter-derived CO 2 emission from Lsoil significantly at day 14 with P =0.02 and P =0.026, respectively. Full size image Earthworm-induced unequal C processes in soil aggregates One of the major ways that earthworms impact C cycling is to regulate the soil aggregation process [9] , [10] . Notably, the aforementioned unequal C processes were also manifested in changes of C distribution among aggregate fractions and in the respective humification intensity (soil organic matter gradually becomes 15 N-enriched as humification proceeds; ref. 23 ) ( Fig. 4a,b ). In phase I, both earthworm species enhanced the formation of macroaggregates >2,000 μm ( F =7.43, P =0.024), which increased total organic C (TOC) storage and 15 N abundance ( F =73.01, P <0.001) in that fraction. Further, A. agrestis reduced TOC storage in aggregate fractions of 250–2,000 μm ( P =0.001), 53–250 μm ( P =0.037) and floatable particulate organic matter (FPOM) ( P =0.002), but only increased the 15 N abundance in FPOM ( P =0.005). Similarly, L. rubellus reduced TOC storage in fractions of 250–2,000 μm ( P =0.027) and FPOM ( P =0.012), but only produced a non-significant increase of 15 N in FPOM ( P= 0.091). The changing patterns of 15 N abundance suggest that earthworms have limited capacity to enhance the humification (and, thus, the associated mineralization) of highly humified aggregate fractions. As a result, earthworms disrupted the C distribution in aggregates and stored more C in the highly stable macroaggregate fraction [24] . Moreover, A. agrestis only induced slightly higher abundances of 15 N in FPOM than L. rubellus did at a marginally significant level ( P= 0.062), but induced significantly lower TOC content in aggregates of 250–2,000 μm ( P =0.030) and much higher TOC content in macroaggregates of >2,000 μm ( P =0.001) than L. rubellus . These results suggest that the distinct dietary patterns of earthworms induced minimal changes in C mineralization, but more strongly enhanced C stabilization, which may explain why the smallest CO 2 emissions were observed in Asoil at day 54 ( Fig. 3a,b ). 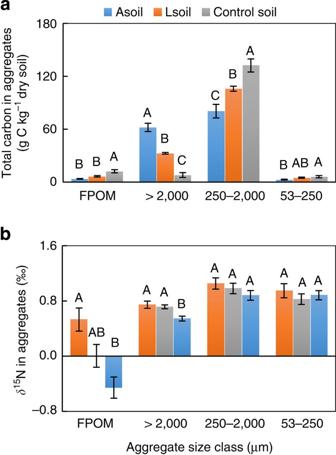Figure 4: Earthworm effects on carbon distribution and humification in aggregates. (a) Carbon distribution and (b)δ15N in phase I. In all panels, mean values are shown±1 s.e.m. (n=3); the s.e.m. is indicated by error bars. The intensity of humification (and concomitant mineralization) is indicated by the natural abundance of15N. Asoil:A. agrestis-worked soil; Lsoil:L. rubellus-worked soil; control soil: sieved field soil which had not been worked with earthworms. FPOM: floatable POM. For a given size class of aggregate, bars with no letters in common are significantly different (P<0.05), whereas those sharing the same letters are not significantly different (P>0.05). Figure 4: Earthworm effects on carbon distribution and humification in aggregates. ( a ) Carbon distribution and ( b ) δ 15 N in phase I. In all panels, mean values are shown±1 s.e.m. ( n =3); the s.e.m. is indicated by error bars. The intensity of humification (and concomitant mineralization) is indicated by the natural abundance of 15 N. Asoil: A. agrestis -worked soil; Lsoil: L. rubellus -worked soil; control soil: sieved field soil which had not been worked with earthworms. FPOM: floatable POM. For a given size class of aggregate, bars with no letters in common are significantly different ( P <0.05), whereas those sharing the same letters are not significantly different ( P >0.05). Full size image Quantifying the unequal C processes To quantify the relative increase in the magnitude of C mineralization and C stabilization and, thus, the change of C sequestration induced by earthworms, we introduce the new concept of sequestration quotient (SQ, C sta /C act ) ( Fig. 1 ). For a system without earthworms, C processes are primarily regulated by soil microbiota; a basal sequestration quotient (SQ basal ) can be calculated as the ratio of microbiota-stabilized C (C sta-m ) to microbiota-activated C (C act-m ). For a system with earthworms, the sequestration quotient (SQ worm ) is calculated as the ratio of earthworm-stabilized C (C sta-w ) to earthworm-activated C (C act-w ). We estimated the values of SQ basal in Lsoil without earthworms and SQ worm in Lsoil with A. agrestis through monitoring the mineralization and stabilization of added 13 C-labelled litter-derived C during phase II. Intriguingly, A. agrestis activated a larger amount of C ( t =−3.04, P =0.039) and stabilized a greater proportion of it ( t =−2.92, P =0.043 for estimation I; t =−4.50, P =0.046 for estimation II; Fig. 5 ), that is, C sta-w exceeded the expected magnitude that may be naturally associated with the increased ingestion and processing of mineralizable C, and, thus, SQ worm exceeded SQ basal ( Fig. 5a ). In this case, earthworms converted a greater proportion of the earthworm-activated C (C act-w ) into the pool of stabilized C (C sta-w ) concomitant with a readily observed increase in CO 2 emission (C min-w ). Importantly, from the aggregates data in the literature [21] , there is strong evidence in support of this logic ( Fig. 5b ; Supplementary Table S1 ). Re-analysis of these data [21] indicates that the endogeic earthworm species ( Aporrectodea caliginosa ) increased both CO 2 emission and sequestration of both TOC and litter-derived C, with SQ basal (0.17) <SQ worm (0.73) <1 and SQ basal (0.02) <SQ worm (0.28)<1, respectively; whereas A. caliginosa increased the sequestration but reduced the mineralization of SOC-derived C, with SQ worm (1.34) >1>SQ basal (0.29). A SQ worm >1, indicating that earthworm-stabilized basal C was greater than earthworm-activated mineralizable C ( Supplementary Table S1 ). 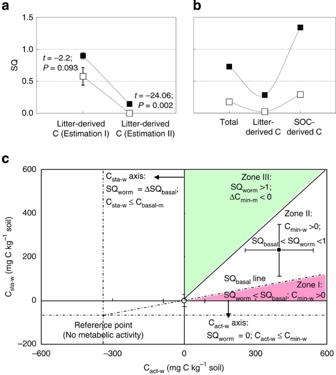Figure 5: Sequestration quotient and its connection with C sequestration. The sequestration quotient (SQ) in phase II (a) and in the literature21(b), and the conceptual diagram (c) showing how to predict the impacts of earthworms on CO2emission and net C sequestration with SQ values. In panels (a,c), means are shown±1 s.e.m.,n=3 in panel (a),n=5 in panel (c); the s.e.m. is indicated by error bars. Earthworms converted the PMC into readily mineralizable C, and protected a larger proportion of readily mineralizable C. SQworm(closed squares) and SQbasal(open squares) values were calculated to quantify the balances between C mineralization and C stabilization in soil with and without earthworms, respectively. Estimation I: all litter-derived C in soil aggregates were assumed to be stabilized; estimation II: about 17% of litter-derived C in microaggregates within large macroaggregates and only 8% of litter-derived C in microaggregates were assumed to be stabilized for soil with and without earthworms, respectively21. In (c) the two dot-dash axes represent the referencexaxis andyaxis in control soil without earthworms; the origin of the dot-dash axes refers to a reference point of no metabolic activity. The two bold grey axes represent thexaxis andyaxis in soil with earthworms, namely the net effects of earthworms on C activation (Cact-waxis) and C stabilization (Csta-waxis); Zones I, II and III indicate the three major scenarios of the contribution of earthworms to C sequestration. The open white circle, that is, the origin of the bold grey axes (Cact-m, Csta-m), refers to the mean values of Cact-mand Csta-min control soils, that is, the basal point. The closed black circle (Cact-w, Csta-w) refers to those values in soils with earthworms. Data are the same as presented in panel (a,b). Csta-mor Cmin-mand Csta-wor Cmin-wrefer to the soil microbiota-induced and earthworm-induced Cstaor Cmin, respectively. As part of Cmin-mmay be metabolized and/or stabilized by earthworms, Cmin-mis also defined as basal C (Cbasal-m). Note that the conversion rate from PMC to Cmin-mand Csta-mmay also be affected by earthworms, thus the value of Cmin-m(Cbasal-m) in a system with and without earthworms may gradually differ as earthworm incubation proceeds. Figure 5: Sequestration quotient and its connection with C sequestration. The sequestration quotient (SQ) in phase II ( a ) and in the literature 21 ( b ), and the conceptual diagram ( c ) showing how to predict the impacts of earthworms on CO 2 emission and net C sequestration with SQ values. In panels ( a , c ), means are shown±1 s.e.m., n =3 in panel ( a ), n =5 in panel ( c ); the s.e.m. is indicated by error bars. Earthworms converted the PMC into readily mineralizable C, and protected a larger proportion of readily mineralizable C. SQ worm (closed squares) and SQ basal (open squares) values were calculated to quantify the balances between C mineralization and C stabilization in soil with and without earthworms, respectively. Estimation I: all litter-derived C in soil aggregates were assumed to be stabilized; estimation II: about 17% of litter-derived C in microaggregates within large macroaggregates and only 8% of litter-derived C in microaggregates were assumed to be stabilized for soil with and without earthworms, respectively [21] . In ( c ) the two dot-dash axes represent the reference x axis and y axis in control soil without earthworms; the origin of the dot-dash axes refers to a reference point of no metabolic activity. The two bold grey axes represent the x axis and y axis in soil with earthworms, namely the net effects of earthworms on C activation (C act-w axis) and C stabilization (C sta-w axis); Zones I, II and III indicate the three major scenarios of the contribution of earthworms to C sequestration. The open white circle, that is, the origin of the bold grey axes (C act-m , C sta-m ), refers to the mean values of C act-m and C sta-m in control soils, that is, the basal point. The closed black circle (C act-w , C sta-w ) refers to those values in soils with earthworms. Data are the same as presented in panel ( a , b ). C sta-m or C min-m and C sta-w or C min-w refer to the soil microbiota-induced and earthworm-induced C sta or C min , respectively. As part of C min-m may be metabolized and/or stabilized by earthworms, C min-m is also defined as basal C (C basal-m ). Note that the conversion rate from PMC to C min-m and C sta-m may also be affected by earthworms, thus the value of C min-m (C basal-m ) in a system with and without earthworms may gradually differ as earthworm incubation proceeds. Full size image According to the changing patterns of C loss and the natural abundance of 15 N in soil aggregates, we ascertained that the C mineralization capacities of earthworms are non-species-specific and no greater than that of soil microbiota alone. This supports our idea that both earthworms and soil microbiota are restricted by the small pool size of PMC. Furthermore, limitation by PMC may partially answer two of the aforementioned questions: why did SOC stocks not decrease when earthworms stimulated increased CO 2 emissions and why did earthworms belonging to different functional groups stimulate similar amounts of CO 2 emissions [5] ? Given that their capacity for C mineralization is similar to soil microbiota and limited ( Fig. 4b ; ref. 5 ), the contributions of earthworms to C sequestration will be determined primarily by their effects on C stabilization. There are three key issues, first, how much C may be activated by earthworms? Second, what proportion of mineralizable C will be metabolized by earthworms (including gut microbiota)? Third, what amount of the earthworm-activated C and basal C could be stabilized by the earthworm-mediated aggregation? Therefore, the pools of basal C (C basal-m ) and PMC and factors, such as soil texture and dietary niches of earthworms that may greatly affect the magnitude of C stabilization, should be considered carefully ( Fig. 1 ). Based on this framework, the relatively slower rates of the earthworm-stimulated CO 2 emissions in rich soil (with high SOC content) seem to be understandable. In a system with low SOC content, both earthworms and microbiota are likely C-limited, with a greater proportion of the earthworm-activated C used to sustain their metabolism, which is quickly lost as CO 2 emissions; therefore, C mineralization may be the dominant process, with less C stabilized. In contrast, in a system with high SOC content, C that is metabolized by earthworms and microbiota may account for a small proportion of a large pool of mineralizable C. Thus, the stimulating effect of earthworms on CO 2 emission is reduced in a relative sense, and C stabilization may be the dominant process. In short, earthworms seem to have different impacts on the ecosystem C cycle, depending on SOC content. Overall, earthworms affect the balance of C mineralization and C stabilization by regulating the size and proportion of three C pools, that is, PMC, readily mineralizable C, and stabilized C ( Fig. 1 ). First, earthworms accelerate the activation of the PMC and the aggregation processes (break up pre-existing aggregates and rebuild new ones), which may stabilize a large proportion of this activated C; simultaneously, part of the unstabilized basal and earthworm-activated C will be mineralized. As a result, both C protected in aggregates (C sta-w ) and stimulation of CO 2 emission (C min-w ) may be directly proportional to the pool of earthworm-activated C (C act-w ). We propose that the patterns of the earthworm-induced CO 2 emission and net C sequestration can be predicted by the difference between SQ basal and SQ worm ( Fig. 5c ). In a system without earthworms, normally SQ=SQ basal <1 (SQ basal line), that is, a small proportion of soil microbiota-activated C (C act-m ) could be protected. In a system with earthworms, earthworms stimulate CO 2 emission but do not affect C sequestration if SQ worm =SQ basal ; earthworms stimulate CO 2 emission and reduce net C sequestration if SQ worm <SQ basal (Zone I); earthworms stimulate CO 2 emission but facilitate C sequestration if SQ basal <SQ worm <1 (Zone II); and earthworms facilitate C sequestration and reduce CO 2 emission if SQ worm >1 (Zone III), that is, the quantity of basal C (C basal-m ) stabilized by earthworms is greater than the quantity of mineralizable C newly activated by earthworms and their gut microbiota. If SQ worm =1 (the dividing line between Zone II and Zone III, Fig. 5c ), earthworms do not change CO 2 emission, but still enhance net C sequestration because large amounts of C, which are equivalent to the entire earthworm-activated C are stabilized by earthworms. Note that on the right part of the C act-w axis, all earthworm-activated C will eventually be mineralized ( Fig. 5c ). A point located on the C act-w axis may represent the extreme situation of soil with low mineralizable C. In contrast, on the upper part of the C sta-w axis, earthworms do not activate C and directly metabolize the basal C (C basal-m ) ( Fig. 5c ). In this situation, earthworms will facilitate C sequestration as long as C sta-w >0, because SQ basal has been increased by earthworms. A point located on the C sta-w axis may represent the extreme situation of soil with high mineralizable C. Our findings indicate that there is an earthworm-mediated ‘C trap’ (ECT) through which regular processes of C sequestration are interrupted, and most of the C flows rapidly into the earthworm gut where it is converted into stabilized forms ( Fig. 6 ). Therefore, earthworms may facilitate C sequestration through an unequal amplification of C stabilization compared with C mineralization. Obviously, CO 2 emission will be damped by the increasing negative feedback effect of the earthworm-induced C stabilization if earthworms stabilize more C than they mineralize; this may partially explain why the earthworm-induced CO 2 emissions decline through time ( Fig. 7 ; ref. 5 ). 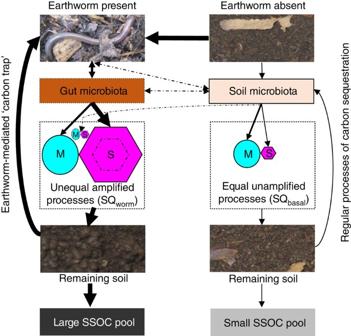Figure 6: Diagram showing the earthworm-mediated carbon trap. The earthworm-mediated ‘C trap’ (ECT) diverted C flow from soil microbiota and unequally enhanced C stabilization and C mineralization. The arrow weight indicates C flow or impact magnitude; single-ended arrow with dotted-line indicates smaller relative effects of soil microbiota when earthworms are present. ‘M’ and ‘S’ represent C mineralization and C stabilization, respectively, their sizes represent the carbon flux of each process, and the dotted-line suggests that the size of the flux can be smaller. SSOC: stabilized soil organic C. ‘Equal unamplified processes’ means each unit of C mineralized naturally along with proportionally less C being stabilized, that is, Csta-mis usually less than Cmin-m, and Csta-mchanges with Cmin-mby a constant range of proportions, resulting in the basal sequestration quotient (SQbasal)<1. ‘Unequal amplified processes’ means small amplification of C mineralization along with great enhancement of C stabilization, that is, Csta-wchanges with Cmin-wby a constant range of proportions, which are usually higher than those in control soil, resulting in the earthworm-induced sequestration quotient (SQworm)>SQbasal. Dotted area and double-ended arrows represent possible interactions. Figure 6: Diagram showing the earthworm-mediated carbon trap. The earthworm-mediated ‘C trap’ (ECT) diverted C flow from soil microbiota and unequally enhanced C stabilization and C mineralization. The arrow weight indicates C flow or impact magnitude; single-ended arrow with dotted-line indicates smaller relative effects of soil microbiota when earthworms are present. ‘M’ and ‘S’ represent C mineralization and C stabilization, respectively, their sizes represent the carbon flux of each process, and the dotted-line suggests that the size of the flux can be smaller. SSOC: stabilized soil organic C. ‘Equal unamplified processes’ means each unit of C mineralized naturally along with proportionally less C being stabilized, that is, C sta-m is usually less than C min-m , and C sta-m changes with C min-m by a constant range of proportions, resulting in the basal sequestration quotient (SQ basal )<1. ‘Unequal amplified processes’ means small amplification of C mineralization along with great enhancement of C stabilization, that is, C sta-w changes with C min-w by a constant range of proportions, which are usually higher than those in control soil, resulting in the earthworm-induced sequestration quotient (SQ worm )>SQ basal . Dotted area and double-ended arrows represent possible interactions. 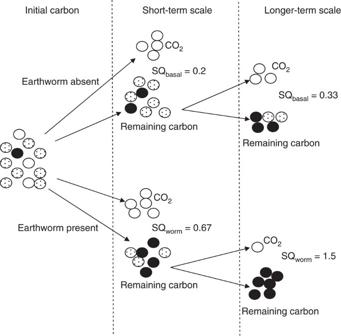Figure 7: Timescale-dependent contrasting effects of earthworms on C sequestration. Conceptualized interpretation of the effect of earthworms on carbon sequestration from an initial state and during short-term and long-term experiments. White symbols: readily mineralizable carbon. Dotted symbols: potentially mineralizable carbon. Black symbols: stabilized carbon; the degrees of shading represent C stabilization accordingly. In most short-term experiments, C mineralization is often stimulated by earthworms, whereas the concomitant C stabilization that may reduce subsequent C mineralization is normally overlooked or hard to detect. Thus, the effect of earthworms on C mineralization is more likely to be overestimated, whereas the earthworm effect on C stabilization is likely to be underestimated. Through the ECT process, C stabilization is enhanced but C mineralization is damped over time, resulting in accumulation of more stabilized C. The values of the sequestration quotient (SQ) reflect the changing patterns of CO2emission and net C sequestration exactly. Therefore, earthworms may be found to protect C at the beginning (over the short time scale), as well as over the long term, when considering both C mineralization and C stabilization. Full size image Figure 7: Timescale-dependent contrasting effects of earthworms on C sequestration. Conceptualized interpretation of the effect of earthworms on carbon sequestration from an initial state and during short-term and long-term experiments. White symbols: readily mineralizable carbon. Dotted symbols: potentially mineralizable carbon. Black symbols: stabilized carbon; the degrees of shading represent C stabilization accordingly. In most short-term experiments, C mineralization is often stimulated by earthworms, whereas the concomitant C stabilization that may reduce subsequent C mineralization is normally overlooked or hard to detect. Thus, the effect of earthworms on C mineralization is more likely to be overestimated, whereas the earthworm effect on C stabilization is likely to be underestimated. Through the ECT process, C stabilization is enhanced but C mineralization is damped over time, resulting in accumulation of more stabilized C. The values of the sequestration quotient (SQ) reflect the changing patterns of CO 2 emission and net C sequestration exactly. Therefore, earthworms may be found to protect C at the beginning (over the short time scale), as well as over the long term, when considering both C mineralization and C stabilization. Full size image The earthworm species studied here and previously [21] belong to the two largest taxonomic groups respectively, that is, Lumbricidae and Pheretimoid, which have spread throughout the temperate and tropical regions of the globe [12] . In addition, most earthworm individuals were alive and healthy in the present study throughout the experiment ( Supplementary Fig. S1 ). Therefore, we think these species are reasonably representative of earthworms in general and suitable for estimating the SQ worm pattern resulting from the ECT process. Given that the values of SQ worm are greater than those of SQ basal ( Fig. 5 ), the ECT process may enhance net carbon stabilization. However, the global contribution of earthworms to soil C storage, and whether the degree of that enhancement would be of a magnitude to have any measurable negative effect on global warming, are still uncertain. First, the pool size of earthworm-stabilized C in the real world is difficult to measure accurately, because its distribution pattern within the whole soil profile and its transfer into other systems, such as ground water and rock strata, are scarcely known. In addition, although C in earthworm casts is more resistant to mineralization than C in control soil [9] , the residence time of earthworm-stabilized C has not been quantified. Second, the difference between SQ worm and SQ basal may vary with earthworm species or ecological groups (that is, epigeic, endogeic and anecic species), soil characteristics (for example, soil texture, SOC content) and plant traits (for example, plant diversity, litter and root C input). In other words, the effects of earthworms on net C sequestration at the ecosystem scale are difficult to quantify in a simple short-term experiment. For instance, earthworms interact with plant species and impact plant productivity of the sites, which feeds back on C sequestration on the time scale of years to decades or more. Thus, it is unlikely that a short duration study can determine the actual amount of carbon being sequestered by earthworms in the field. On the one hand, the earthworm-stimulated CO 2 emission may be partially offset or even overcompensated by C sequestration resulting from plant uptake if net primary productivity increases in response to nutrients released by the accelerated mineralization [12] . On the other hand, plant productivity may be reduced and, thus, feedback negatively on the amount of carbon that earthworms can sequester if a significant proportion of the nutrients that earthworms liberate from leaf litter or SOC is leached away. Third, different disturbances or land uses may exert contrasting effects on earthworm biomass and thus their contribution to C sequestration. Given that C stabilization is likely to increase with earthworm biomass, a greater contribution of earthworms to C sequestration is expected due to the on-going expansion of exotic earthworms into new habitats and increased applications of organic farming. However, increases in extreme weather events and global soil degradation, and their negative effects on earthworm populations, may reduce earthworm contributions to C sequestration. Nevertheless, the SQ-based conceptual model proposes a quantitative approach to understand the process by which earthworms impact C sequestration. The global contribution of earthworms to C cycling may be clearer when the ranges of SQ worm and SQ basal have been determined at different time-scales in a range of systems with variable environmental characteristics (for example, climate, plant diversity, root C input, soil texture and food-web structure). Much attention has been paid to earthworms during the last few decades, during which some invaded species were found reducing forest floor considerably in North America [25] . One of the possible results of the significant loss of forest floor is that much more C will be stored within soil in more stabilized forms because litter C may be transported into soil and stabilized by the aggregation processes ( Fig. 6 ; Supplementary Fig. S2 ). A recent field experiment in North American forests also indicates that earthworms convert PMC into readily mineralizable carbon and stabilized carbon simultaneously [26] . Further, although only part of the earthworm-incorporated litter C in soil (for example, C in the microaggregate within macroaggregate fraction) may be stabilized, the earthworm-stabilized carbon may accumulate during the conversion progress of PMC [21] , [26] . Nevertheless, whether earthworms enhance or reduce the net stabilization of TOC in those North American forests is unknown because only the stability of the incorporated 13 C-labelled litter C has been examined, whereas the stability of earthworm-worked SOC has not been quantified in the field. Perhaps, earthworms are special mobile ‘hotspots’ of soil biogeochemical cycling, which contribute positively to the two contrasting important ecosystem services of nutrient cycling and C sequestration simultaneously. The present study introduces a methodology to understand the ecological processes through which earthworms may facilitate C sequestration (and related nitrogen and phosphorous cycling). Further studies are needed, however, to address the aforementioned uncertainties in earthworms’ contribution to net C sequestration so that the generality, threshold value, and duration of the ECT process can be better estimated. Such information is critical for the prediction and management of the carbon cycle at both local and global scales. Experimental configuration A two-phase microcosm experiment was conducted. Phase I was an incubation of sieved and homogenized forest soil with or without earthworms for 23 days. Thus, the effects of earthworms on soil C loss, humification intensity (which was indicated by increasing 15 N natural abundance; ref. 23 ) and C stabilization (aggregates formation) were investigated. In addition, three different soil treatments, that is, Amynthas -worked soil (Asoil), Lumbricus -worked soil (Lsoil) and control soil incubated without earthworms (control soil) were obtained. In phase II, the three soil treatments plus 13 C-labelled oak litter were incubated with or without earthworms for an additional 31 days. To test the hypothesis that the C mineralization capacity of earthworms is no greater than that of soil microbiota, C losses from treatments with earthworms in phase I and from earthworm-removed earthworm-worked soils (that is, Asoil and Lsoil) in phase II were compared with those from control soil. To evaluate the relative contributions of earthworms to C mineralization and C stabilization, the CO 2 emission rates of earthworm-removed Asoil and Lsoil were compared with those of control soil when the SOC content had declined to similar levels (that is, day 54); furthermore, the sequestration quotients (SQ, C sta /C act ) in treatments with (SQ worm ) and without earthworms (SQ basal ) were calculated to reflect and predict the effects of earthworms on CO 2 emission and C sequestration according to measurements of 13 C abundances in CO 2 and soil aggregates (ref. 21 ). Phase I experiment Phase I represents a common microcosm study of earthworm incubation. Soil (0–5 cm) and earthworms were collected from a ~2 km 2 area on the western edge of the Great Smoky Mountains National Park (35°31′30′′–35°33′27′′ N; 83°59′35′′–84°00′36′′ W). Detailed descriptions of soil and vegetation at the field site are provided elsewhere [22] . Nine samples of field soil were collected and freeze-dried for measurements of stable isotope ratios ( δ 15 N and δ 13 C) and SOC content. Soil was sieved (2 mm), air-dried and mixed to create a homogenous substrate. Thirty experimental units were made using polyvinyl chloride pipes (15 cm in height, 10.4 cm in diameter) and cleaned with 75% ethanol. Two hundred grams of air-dried soil was added to each microcosm and soil water content was adjusted to 60% of the maximum water-holding capacity. Each microcosm was weighed every 3 days and water added to maintain constant moisture content; room temperature was maintained at 18 °C. After 1 week of static culture, 12 microcosms were inoculated with A. agrestis (three individuals per microcosm); another 12 microcosms with L. rubellus (three individuals per microcosm) and the remaining 6 were incubated as controls without earthworms. Given that earthworms seem to show an aggregate distribution, a relatively high population density of earthworms (approximately 353 ind. m −2 ) was used to make it easier to detect the effects of earthworms on C cycling through a short-term incubation. The initial earthworm biomass in each microcosm was recorded and 0.1 g non-labelled oak litter was placed on the surface of each microcosm. After 23 days of incubation, three microcosms from each treatment were randomly chosen and destructively sampled. Earthworms of each microcosm were weighed again. One hundred sixty-five grams of soil was collected from the three replicates of each treatment and then air-dried for 1 week [27] . Fifty grams of dried soil from each sample was then wet-sieved to determine aggregate size distribution [28] ; a sample of each aggregate fraction was weighted for stable isotope ( 13 C and 15 N) and SOC content analyses. An aliquot of each earthworm and soil sample was freeze-dried for stable isotope and SOC content analyses. Earthworms were removed by hand from the remaining 21 microcosms and grouped by species. Each treatment of soil (Asoil, Lsoil and control soil) was mixed thoroughly. All remaining earthworms and soils were kept for the phase II experiment. Phase II experiment During phase II, earthworms were re-introduced. The three treatments of soil were incubated with or without earthworms for an additional 31 days. The seven treatments (each with three replicates) were: three individuals of A. agrestis in Asoil, three individuals of A. agrestis in Lsoil, three individuals of L. rubellus in Lsoil, three individuals of L. rubellus in Asoil, Asoil without earthworms, Lsoil without earthworms, and the control soil without earthworms. As in phase I, 200 g equivalent of dry soil was added to each microcosm, and soil water content was adjusted to the initial level. Every 3 days, each microcosm was weighed, and water was added to maintain constant moisture content. Room temperature was also maintained at 18 °C. Before experiment initiation, the microcosms were static-cultured for 2 days. Earthworms were then inoculated into microcosms after 1 day of gut-voiding on wet filter paper, and 1 g autoclaved (121 °C, 30 min) 13 C-enriched oak litter (~4 mm size, δ 13 C=453.97±15.66‰, δ 15 N=2.37±0.02‰) was placed on the soil surface. After 31 days of incubation, the litter on the soil surface in some microcosms with L. rubellus was almost gone, so the experiment was terminated. All microcosms were sampled destructively. A subsample of bulk soil from each microcosm was freeze-dried for stable isotope and SOC content analyses. Earthworm numbers in each microcosm were recorded and earthworm biomass was measured after 1 day of gut-voiding. Earthworms were then euthanized by placement in a freezer (−20 °C) for 2–5 min, the posterior 33% of the body was removed, and the gut was cleaned with deionized water and freeze-dried for isotope and C content analyses. The anterior 67% of each earthworm was preserved in 70% ethanol for confirmation of taxonomic identity. Dried subsamples of about 13 mg of soil, 1.5 mg of earthworm tissue and 6 mg of litter were used for analysis of stable C and N isotope ratios with an Elemental Analyser/Thermo-Finnigan Delta Plus IRMS (Thermo Scientific, Bremen, Germany) in University of Georgia, GA, USA. Measurements to determine the mineralization patterns of litter- and SOC-derived C were begun after 3 days of static culture of earthworm. Four tests of CO 2 flux were performed with an interval of 4–10 days (that is, on July 3, July 13, July 23 and July 30). A septum was added to the top of each microcosm to form a sealed headspace (539±1.6 ml). Gas samples were collected using a gas-tight syringe from the headspace via the septum. Each microcosm was covered and 20 ml of gas was collected and transferred to an evacuated 12 ml glass tube (Exetainer, Labco) at zero time and 1 h later. A 5 ml aliquot of gas was taken from each tube for 13 CO 2 analysis. A 1 ml aliquot of gas was used to measure the CO 2 concentration of each sample with a Carle AGC 100 GC (EG&G Chandler Engineering, Tulsa, OK, USA) equipped with a thermal conductivity detector at the USEPA in Athens, GA. C fluxes Total CO 2 flux was calculated according to the following equation: where C(t) total is the total hourly flux of CO 2 of each microcosm (mg C h −1 ), d c /d t is the change in CO 2 concentration during the 1 h incubation ( v / v , p.p.m. per hour), M is the molecular weight (mg mmol −1 ) of CO 2 expressed in terms of C, T is the incubation temperature in degrees Kelvin (K), T 0 is standard temperature in degrees Kelvin (K), V 0 is the molar volume of CO 2 under standard conditions (22.4 ml mmol −1 ), and V represents the volume of the headspace (ml). Standard atmospheric pressure was assumed for these calculations. A three-source mixing model was used to partition litter and SOC-derived CO 2 flux for the four tests [29] and these results were used to estimate the cumulative litter- and SOC-derived CO 2 fluxes in phase II. The equations of the three-source mixing model are: and where f t0 is the fraction of the background CO 2 mass to the total CO 2 amount at the end of 1 h incubation, f litter and f soc are fractions of litter and SOC-derived CO 2 , respectively; δ 13 CO 2−t0 and δ 13 CO 2−t1 represent 13 C abundance of CO 2 at zero time and 1 h later, respectively; δ 13 C litter and δ 13 C soc are 13 C abundance of the labelled oak litter and the 23 day-incubated soil, respectively, with or without earthworms. Subsequently, litter and SOC-derived CO 2 flux during the four tests were calculated by combining equation1 to 3, and cumulative litter or SOC-derived CO 2 flux was calculated according to the equation: where C ( t ) is the cumulative litter or SOC-derived CO 2 flux, C ( t i ) and C ( t i +1 ) represent litter or SOC-derived CO 2 flux during the four tests, d is the interval days between a given two tests with i changing from 0–3, C ( t 0 ) is assumed to be the same as C ( t 1 ). A three-source mixing model was used to calculate litter or SOC-derived carbon in earthworm biomass during the 31 days experiment. The equations are: and where f b is the earthworm background carbon fraction, which was assumed to be 0.75 as the experimental duration was short [22] , Δ represents the enrichment factor of earthworms from their putative diets, which was assumed to be 3.68‰ (ref. 22 ), f litter’ and f soc’ are fractions of litter and SOC-derived carbon, respectively, in earthworm biomass at the end of the 31 day incubation; δ 13 C worm−t0 and δ 13 C worm−t1 represent 13 C abundance of earthworms at the zero time and 31 days later, respectively; δ 13 C litter and δ 13 C soc are the same as in equation 3. The total litter and SOC-derived carbon in earthworm tissues were then calculated with the combination of data such as earthworm biomass, water content (assumed to be 0.75) and earthworm carbon content. A simple mixing model was used to calculate the fraction of litter-derived carbon in soil [30] . The equation used was: where f litter′′ is the fraction of litter-derived carbon in soil, δ 13 C soc−t0 and δ 13 C soc−t1 are 13 C abundance of SOC at zero time and at the end of the 31 days experiment, respectively, δ 13 C litter is 13 C abundance of the same labelled oak litter. The total litter-derived carbon in soil was then calculated by combining the data of total SOC content. Calculations of SQ worm and SQ basal In phase II, given that A. agrestis stimulated CO 2 emission only in L. rubellus -worked soil (Lsoil), we analysed both the cumulative 13 C-labelled litter-derived CO 2 emission (C min ) and the litter-derived C in soil aggregates (C sta ) for Lsoil. Thus, the sequestration quotients in Lsoil with A. agrestis (SQ worm ) and without A. agrestis (SQ basal ) were estimated. Soil aggregates (50 g dry weight) were separated into three fractions, that is, large macroaggregate >2,000 μm, small macroaggregate 250–2,000 μm, and microaggregate 53–250 μm. Total C and 13 C abundance in each aggregate fraction were measured. Estimation I. Given that litter-derived CO 2 in soil with or without A. agrestis decreased to a low level after 14 days ( Fig. 3b,d ), upper-bound estimates of SQs can be obtained by assuming that all of the litter-derived C in soil aggregates was stabilized. Thus, C stabilization (C sta ) was equal to the sum of litter-derived C in all the three fractions of aggregates; the fraction of litter-derived C in each aggregate fraction was calculated with equation 7. The value of SQ basal was then calculated as: C sta-m and C min-m refers to the basal C sta and C min , respectively, in soil without earthworms (that is, Lsoil without A. agrestis ). C sta-w and C act-w are the differences of C sta and C act between soil with and without earthworms, respectively; C sta and C act refer to the directly measured pool of stabilized C and the pool of stabilized C plus readily mineralizable C, respectively. C sta-m and C min-m refer to the average of pools of the stabilized C and readily mineralizable C, respectively, for the three replicates of Lsoil without A. agrestis . Estimation II. The C stabilization (C sta ) was likely overestimated if all litter-derived C in aggregates was assumed to be stabilized as in estimation I, especially for Lsoil without A. agrestis (C sta-m ). According to the data in the literature [21] , about 8% of the litter-derived C in microaggregates of 53–250 μm and 17% of that in large macroaggregates of >2,000 μm (as microaggregate within large macroaggregates) were stabilized for the control soil and earthworm-treated soil, respectively. Thus, C sta-m =8% (litter-derived C in microaggregate), and C sta-w =17% *(litter-derived C in large macroaggregates). C min-m and C min-w were the same as that in estimation I. The SQ basal and SQ worm were then calculated with equation 8 and equation 9, respectively. Similarly, the SQ basal and SQ worm for TOC, 13 C-labelled litter-derived C and SOC were calculated with equation 8 and equation 9, respectively, and data from the literature (ref. 21; Supplementary Table S1 ). Statistical methods A one-sample t- test (two-tailed) was performed to examine the impacts of earthworms and soil microbiota on the carbon loss pattern during the two-phase experiment ( Fig. 2 ). One-way ANOVA was performed to compare the differences between total SOC content among the control soil and the earthworm-removed earthworm-worked soils (that is, Asoil and Lsoil) at the end of the two-phase experiment ( Fig. 2 ); to examine the effect of earthworms or the earthworm-worked soils on the SOC- or litter-derived CO 2 emissions during phase II ( Fig. 3 ); to examine the effects of earthworms on the organic carbon content and the natural abundance of 15 N in different fractions of soil aggregates ( Fig. 4 ); and to examine the effects of earthworms on the allocation of the litter-derived C into earthworm biomass, soil and air ( Supplementary Fig. S2 ). A repeated measures ANOVA was performed to compare the effects of the two earthworm species on SOC- or litter-derived CO 2 flux during phase II (data from Asoil and Lsoil were pooled together) ( Fig. 3c,d ). Independent-sample t- tests (two-tailed) were performed to compare the differences between the values of the sequestration quotient (SQ) or the amounts of activated C (C act ) and stabilized C (C sta ) between treatments with and without earthworms ( Fig. 5a ). All statistical analyses were performed with SPSS15.0. How to cite this article: Zhang, W. et al . Earthworms facilitate carbon sequestration through unequal amplification of carbon stabilization compared with mineralization. Nat. Commun. 4:2576 doi: 10.1038/ncomms3576 (2013).